A segmental genomic duplication generates a functional intron An intron is an extended genomic feature whose function requires multiple constrained positions—donor and acceptor splice sites, a branch point, a polypyrimidine tract and suitable splicing enhancers—that may be distributed over hundreds or thousands of nucleotides. New introns are therefore unlikely to emerge by incremental accumulation of functional sub-elements. Here we demonstrate that a functional intron can be created de novo in a single step by a segmental genomic duplication. This experiment recapitulates in vivo the birth of an intron that arose in the ancestral jawed vertebrate lineage nearly half-a-billion years ago. The appearance of a new intron that precisely splits an exon without disrupting the corresponding peptide sequence is a very rare event in vertebrate genomes. No such intron gains have been documented in the human, mouse, rat, or dog lineages since their common mammalian ancestor [1] , nor in a comparison between the pufferfish Fugu and Tetraodon [2] . Nevertheless, a few credible cases of vertebrate intron gain have been documented in teleost fish [3] . In these examples, the novel intron sequences showed recognizable similarity to the surrounding coding exons, and appeared at AG|GT sites embedded within coding sequence. This observation suggested that recent tandem duplication of an AGGT motif-containing coding sequence could have led to the formation of the intron, an idea originally put forward by Rogers [4] . If the 5′-GT and 3′-AG in the duplicated region were recognized by the spliceosome as donor (5′-splice site) and acceptor (3′-splice site) signals, the redundant duplicated region would be excised from the primary transcript, leaving the translated peptide unaltered by the segmental genomic duplication ( Fig. 1 ). 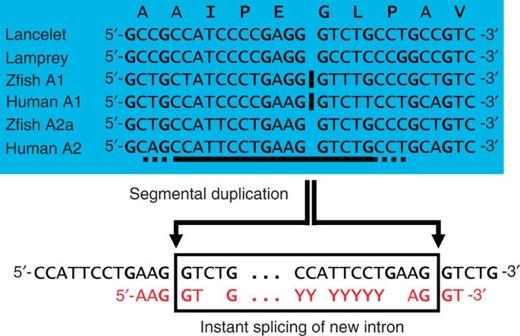Figure 1: Proposed mechanism for intron birth. Extant lancelet and lampreyATP2Agenes, and human and zebrafishATP2A2genes, are intronless in the region shown, reflecting the ancestral chordate condition, but human and zebrafishATP2A1genes are interrupted by an intron between the first and second nucleotides of codon G310 (coordinate with respect to human amino acid sequence ofATP2A1isoform a). The peptide sequence is fully conserved, so only synonymous amino acid codon substitutions are seen in the nucleotide sequence. A segmental tandem duplication encompassing this region would produce a potential intron with consensus donor and acceptor splice sites, including a polypyrimidine tract. The sequence of the intronless humanATP2A2gene is used in this example. Figure 1: Proposed mechanism for intron birth. Extant lancelet and lamprey ATP2A genes, and human and zebrafish ATP2A2 genes, are intronless in the region shown, reflecting the ancestral chordate condition, but human and zebrafish ATP2A1 genes are interrupted by an intron between the first and second nucleotides of codon G310 (coordinate with respect to human amino acid sequence of ATP2A1 isoform a). The peptide sequence is fully conserved, so only synonymous amino acid codon substitutions are seen in the nucleotide sequence. A segmental tandem duplication encompassing this region would produce a potential intron with consensus donor and acceptor splice sites, including a polypyrimidine tract. The sequence of the intronless human ATP2A2 gene is used in this example. Full size image Here we apply a bioinformatic approach to look for early vertebrate-specific intron gains. In addition to the requirement that the intron be absent in invertebrate orthologues, we require that paralogues from the whole-genome duplications at the base of vertebrate evolution contain examples of genes with and without the intron. We find only one example of such an intron gain, namely within the ATP2A family, where an intron is present in the human ATP2A1 gene, but not in ATP2A2 . We test the segmental duplication scenario by creating artificially duplicated constructs of the intronless gene and demonstrate in live human cells that the redundant region can be spliced out, in essence reenacting a plausible creation mechanism for the intron in the ATP2A1 gene. Discovery of the vertebrate-specific ATP2A1 intron gain We conducted a genome-wide search for pairs of human paralogues indicated by conserved synteny to have originated in one of the early vertebrate-specific whole-genome duplications. Such pairs were grouped by sequence similarity with putative orthologues from both vertebrates and invertebrates, and intron splice sites within conserved areas of the coding sequence were identified. Of 252 splice sites that meet strict criteria (Methods) only one, found in ATP2A1, had the signature of a vertebrate-specific gain. The ATP2A gene family encodes sarco/endoplasmic reticulum calcium ATPases (SERCAs) whose dysfunction has been associated with several human diseases [5] . ATP2A genes found outside of the jawed vertebrates are intronless near the motif AAIPE G PLAV, reflecting the ancestral condition ( Fig. 1 ; Table 1 ). Humans and other tetrapods encode three paralogues ATP2A1 , ATP2A2 , and ATP2A3 that encode SERCA1 , SERCA2 , and SERCA3 , respectively. These genes originated from an ancestral chordate gene by two rounds of duplication and subsequent loss of one copy ( Table 1 ; Methods). All vertebrate ATP2A1 genes include a novel intron between the first and second nucleotides of the G310 codon at an AGGT motif ( Fig. 1 ). In contrast, the ATP2A2 and ATP2A3 genes retain the ancestral intronless state at this position. The intron in the ATP2A1 gene splits a single ancestral exon (exon 8 in human ATP2A2) into two exons (exons 8 and 9 in human ATP2A1 ). As the intron is shared by tetrapods and teleost fish, it evidently arose more than 420 million years ago. Table 1 Number of ATP2A genes with and without an intron at the motif AAIPE G LPAV in 15 species. Full size table We can infer much of the ancestral vertebrate ATP2A sequence around G310, because its nucleotide sequence is highly constrained by the perfect conservation of the amino residues, leaving only synonymous coding positions to vary. A segmental duplication containing the AGGT motif contains most of the sequence elements required for recognition by the U2 (major class) spliceosome ( Fig. 1 ). These motifs include several other consensus nucleotides around the donor and acceptor sites [6] ((A/C)AG| GT (A/G)AGT ... .C AG |G) beyond the GT and AG dinucleotides, as well as a polypyrimidine tract (7 of the 8 nucleotides at position −12 to −5 near the acceptor are pyrimidines), and a potential branchpoint A residue with consensus (YTN A Y) at position −48 (not shown). Reenacting the birth of an intron To test the hypothesis that a functional intron can be produced de novo by an appropriate segmental genomic duplication, we designed a mini-gene construct that contains a duplication of ATP2A2 exon 8. The construct was transiently transfected into HEK 293 and HeLa cells, and the resulting messenger RNA characterized. We propose that the duplicated exon 8 in ATP2A2 becomes exons 8 and 9 in ATP2A1 through the creation of a new intron ( Fig. 2a ). The duplicated AGGT motifs span the borders between the exon 8 and 9 regions, and our hypothesis is that the spliceosome will recognize the AG|gt ... ag|GT sequences as splice sites and remove the central exon 9 and exon 8 ( Fig. 2a ). The segmental duplication could be any length, as long as the 5′-GT and 3′-AG are separated by more than the minimal functional intron length, about 60 nucleotides. 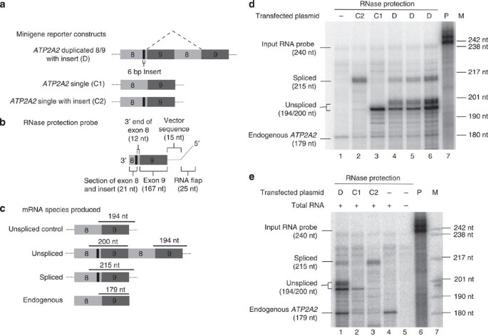Figure 2: Reconstruction of duplicated splice sites undergoes splicing at low levels. (a) Schematic diagram of mini-gene constructs transfected into HEK 293 and HeLa cells includingATP2A2duplicated exon 8/9 (D),ATP2A2Single (C1) andATP2A2Single with 6 bp insert (C2). The sequence corresponding to exon 8 is shaded light grey, exon 9 dark grey, 6 bp insert black and vector sequences are shown by dashed lines. (b) Diagram of the RNase protection probe along with annotations of what sequences each part of the probe will hybridize to. (c) Schematic representation of potential mRNA species from the transfections and the corresponding RNA probe fragments that their presence will lead to in the RNase protection assay. (d) Phosphorimage of RNase protection assay products from HEK 293 cells with DNA size marker sizes (in nt ssDNA) indicated on the right, and what size RNA fragments the protected probe bands correspond to on the left (ssRNA). Transfections were performed in triplicate. (e) Phosphorimage of RNase protection assay products from HeLa cells with DNA size marker sizes (in nt ssDNA) indicated on the right, and what size RNA fragments the protected probe bands correspond to on the right (ssRNA). Transfections were performed in triplicate. Figure 2: Reconstruction of duplicated splice sites undergoes splicing at low levels. ( a ) Schematic diagram of mini-gene constructs transfected into HEK 293 and HeLa cells including ATP2A2 duplicated exon 8/9 (D), ATP2A2 Single (C1) and ATP2A2 Single with 6 bp insert (C2). The sequence corresponding to exon 8 is shaded light grey, exon 9 dark grey, 6 bp insert black and vector sequences are shown by dashed lines. ( b ) Diagram of the RNase protection probe along with annotations of what sequences each part of the probe will hybridize to. ( c ) Schematic representation of potential mRNA species from the transfections and the corresponding RNA probe fragments that their presence will lead to in the RNase protection assay. ( d ) Phosphorimage of RNase protection assay products from HEK 293 cells with DNA size marker sizes (in nt ssDNA) indicated on the right, and what size RNA fragments the protected probe bands correspond to on the left (ssRNA). Transfections were performed in triplicate. ( e ) Phosphorimage of RNase protection assay products from HeLa cells with DNA size marker sizes (in nt ssDNA) indicated on the right, and what size RNA fragments the protected probe bands correspond to on the right (ssRNA). Transfections were performed in triplicate. Full size image The duplicated nature of the construct rendered standard reverse-transcription PCR ineffective at distinguishing between the presence of unspliced and spliced mRNA products from the ATP2A2 duplicated minigene, so we employed RNase protection assays instead. To clearly differentiate spliced from unspliced mRNA, we cloned an extra 6 bp into the 5′ copy of exon 8 near its 3′ end that distinguishes it from the 3′ copy of exon 8 ( Fig. 2a ). The RNase protection probe was designed to take advantage of this small difference between the two exon 8 s ( Fig. 2b ) and will lead to the production of four possible protected RNA probe fragments ( Fig. 2c ). Two control mini-gene plasmids, C1 and C2, were also transfected to act as markers for these predicted RNase protection fragments ( Fig. 2a ). ATP2A2 Single (C1) will give rise to a fragment at the size matching unspliced mRNA from the duplicated construct, 194 nt ( Fig. 2c ). ATP2A2 single with 6 bp insert (C2) will produce a protected fragment corresponding in length to spliced mRNA (215 nt). RNase protection assays were performed with total RNA from the transfections of these three mini-genes along with a no-transfection control and a probe-alone control in HEK 293 cells ( Fig. 2d ) and HeLa cells ( Fig. 2e ). The probe-alone assay leads to the production of low-level non-specific protected fragments, presumably from internal secondary structures in the radiolabelled probe that are RNase resistant ( Fig. 2e , lane 5). The 179 nt protected probe fragment in the no-transfection control ( Fig. 2d , lane 1 and Fig. 2e , lane 4) confirms the presence of endogenous ATP2A2 mRNA transcripts. Our experiments show that segmental duplication can create a functional intron. Using the duplicated ATP2A2 construct, we clearly observed a 215 nt protected probe fragment whose size corresponds precisely to the spliced mRNA control ( Fig. 2d , lanes 2 and 4, 5, 6, and, Fig. 2e , lanes 1 and 3). Quantification of the relative abundance of these protected probe RNA fragments from the ATP2A2 duplication indicates that 15.9% (±1.7%) in HEK 293 cells and 5.9% (±1.2%) in HeLa cells, of the mRNA is spliced. To rule out the possibility that the 215 nt RNase-protection RNA product resulted from rearrangements at the DNA level rather than splicing, plasmid DNA was recovered from HEK 293 cells transfected with the ATP2A2 duplication construct. Characterization of these plasmids with restriction enzyme digestions ( Fig. 3a ) revealed that no such DNA arrangement has taken place ( Fig. 3b ). Although clear evidence for splicing was observed, the majority of protected fragments were 194 and 200 nt, indicating that most of the expressed mRNA was unspliced. Despite the modest level of splicing, we find that the spliceosome can recognize the duplicated splice sites, and that these alone are sufficient to allow the new intron to be excised from mRNA. 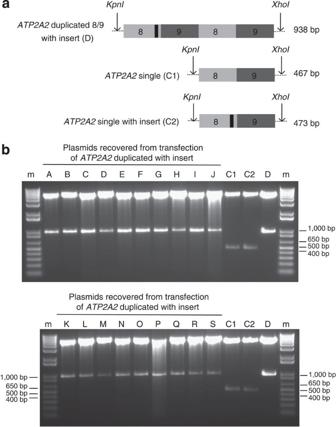Figure 3: Plasmids do not undergo DNA rearrangment during transfection. (a) Schematic of DNA mini-gene constructs used in transfections as described inFigure 2a. Restriction sites are shown along with sizes of DNA digestion fragments. (b) Agarose gels showing diagnostic digests of DNA plasmids recovered from HEK 293 cells transfected withATP2A2duplicated 8/9 with insert (D). Control digests from untransfected plasmids are shown;ATP2A2duplicated 8/9 with insert (D),ATP2A2single (C1) andATP2A2single with 6 bp insert (C2), along with DNA size markers (m). All the recovered DNA plasmids were the same size as the transfected DNA plasmidATP2A2duplicated 8/9 with insert (D). Figure 3: Plasmids do not undergo DNA rearrangment during transfection. ( a ) Schematic of DNA mini-gene constructs used in transfections as described in Figure 2a . Restriction sites are shown along with sizes of DNA digestion fragments. ( b ) Agarose gels showing diagnostic digests of DNA plasmids recovered from HEK 293 cells transfected with ATP2A2 duplicated 8/9 with insert (D). Control digests from untransfected plasmids are shown; ATP2A2 duplicated 8/9 with insert (D), ATP2A2 single (C1) and ATP2A2 single with 6 bp insert (C2), along with DNA size markers (m). All the recovered DNA plasmids were the same size as the transfected DNA plasmid ATP2A2 duplicated 8/9 with insert (D). Full size image The genes of early eukaryotes likely contained many more introns than found in present day eukaryotic genomes, with subsequent genome evolution dominated by intron loss [7] . This suggests an early epoch of massive intron invasion, the mechanism of which has long since been inactivated. In contrast, relatively recent intron gains are very uncommon, particularly within vertebrates. The intron in ATP2A1 discussed in this work is the only example of such an intron gain that we found out of 252 candidate introns within coding regions that are highly conserved across the lancelet, sea urchin, and human genomes (Methods). Such recent intron gains are almost certainly caused by a mechanism different than that responsible for the original genomic invasion of introns [8] . Our results show that a short intragenic tandem duplication can insert a novel U2-type intron into a protein-coding gene, leaving the corresponding peptide sequence unchanged. The novel intron described here was produced by segmental duplication of an AGGT site within coding sequence. Tandem duplications are common in genomes; on the scale of a single gene, Lynch and Conery [9] estimate the order of ∼ 100 gene duplications per genome per million years, and smaller-scale duplications are even more prevalent [10] . The newly created intron is accurately spliced in vivo , albeit at a modest level of ∼ 16% in HEK 293 and ∼ 6% in HeLa cells. The level of spliced mRNA may differ in the fast twitch muscle cells in which ATP2A1 is normally expressed. The splicing efficiency of the originally duplicated sequence of the ancestral vertebrate gene could also have been modulated by synonymous sequence differences relative to our human-genome-based construct, and/or differences in the length and position of the duplicated region. Mutations of the ATP2A1 gene are associated with Brody disease [11] , [12] , an autosomal recessive muscle disorder characterized by impaired relaxation of fast-twitch muscles after excercise. A similar recessive disorder associated with an ATP2A1 mutation has been described in cattle [13] , and the ATP2A1 zebrafish mutant accordion also shows related behavioural defects [14] . The recessive nature of these hereditary disorders implies that vertebrates can tolerate reduced levels of ATP2A1 protein product (SERCA1). Thus, the ancient intragenic tandem duplication that produced the intron-bearing allele in the proto-vertebrate ATP2A1 could have initially spread nearly neutrally through the ancestral population even without 100% splicing efficiency. For the small population sizes characteristic of vertebrates [15] , such an allele could rise to modest frequency and even become fixed, if homozygotes are not at too high of a disadvantage. An allele with 50% splicing efficiency in a homozygous state, for example, would nominally produce the same level of protein product as a heterozygote. Once the intron-bearing allele is fixed, secondary mutations could then emerge to incrementally improve splicing efficiency. The precise gain of an intron as described here is conceptually different from the exon gains previously reported in primates, in which the insertion of ALU elements into existing exons creates a new alternatively spliced exon and adds sequence to the final peptide product [16] . Recruitment of other sequence elements to form or extend exons has also been described [17] . Most other mechanisms for intron gain that have been proposed differ fundamentally from the mechanism documented here, in that they are expected to be accompanied by deletion or insertions within the resulting coding sequence. In contrast, the mechanism we have demonstrated here generates a precisely inserted new intron without any disruption of the surrounding coding sequence. Two examples of probably very recent intron gains have been described in the water flea Daphnia , in which novel introns are still polymorphic in the population [18] . In contrast to the mechanism described here, the newly born introns in Daphnia do not show similarity to flanking (or any known) sequence, and their origin is unknown. This suggests that other intron-creation mechanisms besides the one shown here are also active. Genomewide seach for vertebrate-specific intron gains To identify 'ohnologues', that is, pairs of human paralogues, probably originated in a whole-genome duplication, we assigned position IDs to all loci in the genome, numbering them in the order in which they occur. We used the ENSEMBL models version 55, longest transcript at each locus, and aligned the corresponding 23,266 peptides to each other using BLASTp [19] with an e -value cutoff of 10 −20 . We next identified tandem expanded families, here defined as clusters of neighbouring genes with peptide similarity, allowing a maximum of two intervening genes on any strand. Such clusters were reduced by retaining only the gene with the longest transcript. Genes with strong ( e -value<10 −20 ) similarity to more than twenty other genes (after removing tandem duplicates) were also eliminated to avoid confounding effects of large gene families such as zinc-finger, kinases, or olfactory receptors. Next, we identified pairwise reciprocal highest scoring hits between the remaining genes, restricting further analysis to pairwise hits with scores of at least 60% of that of the maximum of each of the members' reciprocal best hit scores. This left us with 9,852 loci that were re-numbered in strict consecutive orders. We implemented an algorithm similar to that described by Blanc et al . [20] to detect clusters of adjacent genes with sequence similarity to clusters elsewhere in the genome. The mapping of each such gene to its counterpart in the other cluster can be visualized as rungs in a ladder, defining blocks of conserved synteny. To account for the considerable scrambling of gene order by large-scale inversions during half a billion years of evolution, we allowed up to 15 intervening genes between any two rungs. Furthermore, we required each block to contain at least 5 pairs of genes. This analysis resulted in 153 blocks of intragenomic conserved synteny containing a total of 1,007 duplicated pairs of paralogues. These are all expected to be bona fide ohnologues; identical analysis on randomly scrambled gene IDs yielded no false positives. As we aimed to identify early vertebrate intron gains, we chose two outgroups to the vertebrates, namely the Florida lancelet Branchiostoma floridae (a chordate) and the purple sea urchin Strongulucentrotus purpuratus (an echinoderm). For the lancelet, we used the gene annotation by JGI [21] , and, for the sea urchin, the NCBI gene build 2. Reciprocal highest-scoring BLASTp hits yielded 8,501 candidate orthologues between the lancelet and the sea urchin. If both genes in such a pair had mutual best hits to the same human gene, or the same above identified duplicated paraloguous pair, we defined a BHHS (lancelet—human 1—human 2—sea urchin) cluster of orthologues. In total, 426 such clusters were defined. Multiple sequence alignments of the BHHS peptide clusters were performed using clustalW [22] . From these alignments, we extracted gap-free regions flanked by fully conserved amino residues and with no stretch of more than five non-conserved amino residues using custom PERL scripts. The positions and phases of all intron splice sites within such blocks were mapped, and we retained only splice sites flanked by regions with at least six of eight amino residues fully conserved. Finally, we excluded from the analysis sites within 4 amino residues from a non-overlapping splice site in another species, because such cases are mostly caused by gene models with inaccurate intron-exon boundaries. A total of 252 intron splice sites met these stringent criteria. These were evaluated against the wider set of species shown in Table 1 . The signature of a post-duplication vertebrate intron gain would contain a splice site in only one of the two human copies and none of the invertebrate orthologues. In the set examined, we found only a single candidate: the eighth intron in the ATP2A1 gene is absent in all invertebrate orthologues examined, as well as vertebrate paralogues ATP2A2 and ATP2A3 . The distribution of genes with and without this intron in amniotes and telesost fish strongly suggests that this intron gain happened between the two rounds of whole-genome duplication at the base of vertebrate evolution ( Table 1 ). RNase protection assays Mini-gene reporter constructs were generated using genomic PCR of the ATP2A2 gene and cloned into pcDNA3.1 (Invitrogen) between KpnI and XhoI sites (5′-ggcggtggtaccggtacaaacattgctgctgg-3′; 5′-ggcggtctcgagcctgcagactgacatctgg-3′). Overlapping PCR was used to generate the ATP2A2 duplication from ATP2A2 (5′-aaccagatgtcagtctgcaggggtacaaacattgctgctgg-3′; 5′-cctgcagactgacatctgg-3′) and quick-change mutagenesis was employed to insert the extra 6 bp into exon 8 (5′- ccctggctgtagcaggtgattccattcctgaaggtc-3′; 5′-gaccttcaggaatggaatcacctgctacagccaggg-3′). HEK 293 and HeLa cells were grown in standard conditions in DME medium with 5% fetal calf serum. HEK 293 cells (1.5×10 5 ) were transfected with 4 μg DNA Lipofectamine 2000 (Invitrogen). 0.3 μg plasmid DNA was tranfected into 2×10 5 HeLa cells using Effectene (Qiagen). Cells were collected after 48 h and total RNA purified using RNAeasy mini kits (Qiagen). 20 pmol of 32 P-labelled RNA probe, transcribed with T7 polymerase from a PCR fragment generated from ATP2A2 single with insert (5′-ccctggctgtagcaggtg-3′; 5′-taatacgactcactatagggatgtcctttcgctcgacgtcacccctctagactcgagcctg-3′), was hybridized to 10 μg total RNA at 45 °C for 16 h. After cooling to 4 °C, the RNA was incubated with RNases A and T1 at room temperature for 60 min. Following proteinase K treatment, phenol/choloform extraction and ethanol precipitation, protected RNA fragments were resuspended in formamide dyes and run out on 6-8% denaturing polyacrylamide gels. The resulting dried gels were exposed to a phosphorimager screen and bands were quantified with ImageQuant (GE Healthcare). Detailed explanation of RNase protection assay The design of the probe and the duplicated polymorphic construct will lead to the production of four possible protected RNA probe fragments ( Fig. 2c ). Two of these will be protected in the presence of unspliced mRNA at 194 nt (21+12+167 nt) and 200 nt (12+167+15 nt) ( Fig. 2c ). However, if any ATP2A2 duplicated mRNA is spliced, it will hybridize to the probe in such a way as to protect a larger fragment, at 215 nt (21+12+167+15 nt). The presence of endogenous ATP2A2 mRNA, with no intron present will lead to production of a 179 nt fragment (12+167 nt). At the 5′ end of the RNA probe is a section of probe sequence that is not complementary to any ATP2A2 sequence and, therefore, will be digested by the RNases. Its presence creates a difference in protection fragment length between the input probe (240 nt) and the potential protection fragments, allowing confirmation that RNase treatment is working ( Fig. 2d , lane 7 and Fig. 2e , lane 6). Sequences. Exon 8 sequence is shown in bold; exon 9 sequence in standard typeface; 6 bp insert is in italics; vector sequence is dashed underlined; RNA flap sequence is double underlined and T7 promoter sequence is single underlined. DNA sequence of ATP2A2 duplication construct with insert. Recovery of plasmids from transfected cells Plasmid DNA was extracted from transfected HEK 293 cells and transformed into bacteria [23] . From here, they were purified with minipreps (Fermentas) and underwent restriction enzyme digests. The resulting DNA fragments were separated on agarose gels. How to cite this article: Hellsten, U. et al . A segmental genomic duplication generates a functional intron. Nat. Commun. 2:454 doi: 10.1038/ncomms1461 (2011).